Symmetry breaking and optical negative index of closed nanorings Metamaterials have extraordinary abilities, such as imaging beyond the diffraction limit and invisibility. Many metamaterials are based on split-ring structures, however, like atomic orbital currents, it has long been believed that closed rings cannot produce negative refractive index. Here we report a low-loss and polarization-independent negative-index metamaterial made solely of closed metallic nanorings. Using symmetry breaking that negatively couples the discrete nanorings, we measured negative phase delay in our composite ‘chess metamaterial’. The formation of an ultra-broad Fano-resonance-induced optical negative-index band, spanning wavelengths from 1.3 to 2.3 μm, is experimentally observed in this structure. This discrete and mono-particle negative-index approach opens exciting avenues towards symmetry-controlled topological nanophotonics with on-demand linear and nonlinear responses. The theory of diamagnetism was established more than one and a half centuries ago by Weber [1] . At the atomic level, an orbiting current around the nucleus produces microscopic magnetic fields resulting in the magnetism of materials. However, the magnetic relaxation time of orbiting electrons is much longer than the period of optical waves, diminishing the magnetism of natural materials at optical frequencies [2] . Inspired by the atomic orbiting current, metallic closed-ring structures were considered for artificial magnetic responses arising from the induced circulating current. The weak diamagnetism of the closed-ring structures prevents them from having effective permeability below zero, and hence negative indices of refraction [3] . By opening a small gap, the split-ring resonator exhibits a negative permeability due to the significantly enhanced inductance–capacitance resonance. The combination of split-ring resonator with the Drude response from an array of continuous metallic wire into a two-element system led to the first negative index material (NIM) at microwave frequencies and the rapidly emerging field of metamaterials [4] , [5] , [6] , [7] , [8] , [9] , [10] , [11] . However, the long-standing question of the possibility to obtain negative magnetic permeability and negative refractive index with an ensemble of single-element closed rings has remained. Artificial materials, through the engineering of meta-atoms of micro- and nano-structures, have exhibited electromagnetic properties that are not accessible in naturally occurring materials, such as negative refraction [4] , [5] , superlensing [6] , [7] , [8] , electromagnetic cloaking [9] , [10] and unique topological effects [11] . Significant efforts have been devoted to scale NIMs down to the optical domain. The fishnet of metal-dielectric multilayers is one of the most successful optical NIM structures [12] , [13] , [14] , [15] , [16] . The magnetic responses of such structures result from the excitation of gap surface plasmons, and the electrical responses are governed by the cut-off frequency of the waveguide mode of the air holes, resulting in negative-phase index [15] , [16] . Another interesting NIM approach using coupled metal–insulator–metal waveguides has been demonstrated and theoretically extended for broad-angle operation [17] , [18] . Both approaches however rely on continuous metallic structures to form coupled waveguide modes. Here, we experimentally demonstrate optical negative index in a metamaterial that is solely made of closed and discrete metallic nanorings. This is achieved by a subtle symmetry breaking of their arrangement in space. Using a Michelson interferometer, negative-phase delay is directly observed in such a metamaterial, confirming the proposed single-component strategy. The symmetry breaking allows the nanorings to negatively couple to each other and leads to a polarization-independent optical negative index, with extremely broadband from 1.3 to 2.3 μm in the metamaterial. This discrete and mono-particle negative-index approach opens exciting avenues towards isotropic negative-index metamaterials, the key for practical applications. Theory and design of closed nanoring chess metamaterial Discrete metallic nanorings have been studied in rather simple configurations as plasmonic resonators, but have not been able to produce negative permeability or negative indices [2] , [3] , [19] , [20] . We instead consider two layers of coupled rings as schematically shown in Fig. 1a . The localized mode under consideration is the symmetric dipolar mode with charge distribution of the same sign at the inner and outer surface of the ring walls ( Fig. 1b ). Plasmon interactions can be comprehensively described using the analogy with the hybridization of wavefunctions in quantum systems [21] , [22] . The coupling between plasmonic nanorings lifts the degeneracy of the single-particle mode and gives the antisymmetric ( ω − ) and symmetric ( ω + ) modes with magnetic and electric dipole moments, respectively. Symmetric modes have their current flowing in phase in the two rings, whereas for the antisymmetric modes, the currents oscillate out of phase ( Fig. 1b ). The frequency split Δ ω = ω + −ω − = κω 0 is proportional to the coupling coefficient κ . The coupling coefficient between longitudinally coupled electric dipoles is usually positive, and therefore ω + corresponds to the higher energy antibonding mode and ω − to the lower energy bonding mode. When the spatial symmetry of the coupled nanorings is broken as illustrated in Fig. 1a , that is, the rings are sufficiently shifted (by at least dx = dy > L /2, where L is the length of the dipole moment of the single ring), the mode dispersion undergoes a dramatic change due to the modification of the near-field Coulomb interaction, leading to an inversion of the plasmon hybridization scheme. While maintaining charge distribution, an initially bonding mode with magnetic dipole moment when the rings are aligned now becomes antibonding, resulting from symmetry breaking ( Fig. 1b ). The ordering of the modes after symmetry breaking changes the sign of Δ ω and thus corresponds to negative coupling between the nanorings ( Supplementary Fig. S1 ). We show that a three-dimensional (3D) metamaterial built from such negatively coupled discrete rings leads to a negative index and we term it the ‘chess metamaterial’. 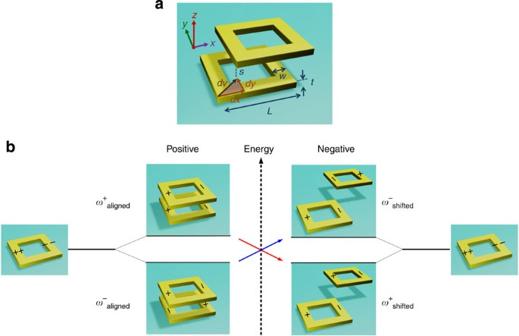Figure 1: Symmetry-dependent hybridization scheme of the closed nanorings. (a) Schematic of the coupled closed nanorings chess metamaterial. (b) Hybridization scheme of the metallic nanorings, depending on their alignment.ω+andω−are the symmetric and antisymmetric modes with electric and magnetic dipole moments. The couplingκbetween the nanorings is defined by Δω=ω+−ω−=κω0, whereω0is the dipole transition of uncoupled or single nanorings. When the rings are aligned (dx=dy=0), the antisymmetric mode corresponds to the bonding mode and occurs at lower energy than the symmetric mode,ω−aligned<ω+aligned. The coupling between the nanorings is positive. When the nanorings are shifted withdx=dy=L, the antisymmetric mode now corresponds to the antibonding mode and occurs at higher energy than the symmetric mode,ω−shifted>ω+shifted, the hybridization is inverted and the coupling between the nanorings is negative. The change in the mode ordering is due to the modification of the near-field Coulomb interaction between the nanorings, where symmetry breaking changes the sign of charges in close interaction. The symmetric (antisymmetric) mode continuously red (blue) shifts with symmetry breaking. Figure 1: Symmetry-dependent hybridization scheme of the closed nanorings. ( a ) Schematic of the coupled closed nanorings chess metamaterial. ( b ) Hybridization scheme of the metallic nanorings, depending on their alignment. ω + and ω − are the symmetric and antisymmetric modes with electric and magnetic dipole moments. The coupling κ between the nanorings is defined by Δ ω = ω + − ω − = κω 0 , where ω 0 is the dipole transition of uncoupled or single nanorings. When the rings are aligned ( dx = dy =0), the antisymmetric mode corresponds to the bonding mode and occurs at lower energy than the symmetric mode, ω − aligned < ω + aligned . The coupling between the nanorings is positive. When the nanorings are shifted with dx = dy =L , the antisymmetric mode now corresponds to the antibonding mode and occurs at higher energy than the symmetric mode, ω − shifted > ω + shifted , the hybridization is inverted and the coupling between the nanorings is negative. The change in the mode ordering is due to the modification of the near-field Coulomb interaction between the nanorings, where symmetry breaking changes the sign of charges in close interaction. The symmetric (antisymmetric) mode continuously red (blue) shifts with symmetry breaking. Full size image Fabrication and experiment We fabricated two layers of shifted gold nanorings on quartz substrates with planarized SU-8 photoresist as spacer. Multiple electron beam lithography processes were employed for the alignment between the layers [22] , [23] . An oblique view of the aligned nanorings structure is shown in Fig. 2a . For shifted nanorings, an equal amount of lateral shift, that is dx = dy , in the transverse plane is used, and results in metamaterials completely insensitive to the incoming polarization at normal incidence, a property crucial for device applications. This was confirmed by polarization-resolved measurements, presented in Supplementary Figs S2–S5 , and so the chess metamaterial properties can thus be probed with unpolarized light. We note that polarization-independent fishnet metamaterials have also been reported [24] , [25] . 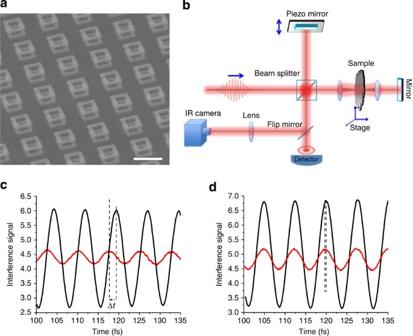Figure 2: Interferometric measurements of the broken symmetry coupled nanorings. (a) Tilted-view scanning electron microscopy image of a metamaterial made of two aligned nanoring layers (dx=dy=0 nm). The scale bar represents 500 nm. (b) Schematic of the Michelson interferometer. The metamaterial under test is made of two layers of nanorings, shifted with respect to each other (dx=dy=L). The thickness (index) of our metamaterial and reference isdmeta(nmeta) anddref(nref), respectively. The time delay between the two corresponding interferograms is related to the index of the metamaterial bynmeta=1+c0Δt/2dmeta+(nref−1)dref/dmeta(Supplementary Fig. S6), wherec0is the speed of light in vacuum. After planarization, the thickness of the metamaterial isdmeta=110 nm and the thickness of the reference on the same substrate isdref=80 nm (nref=1.5). The chess metamaterial being polarization independent at normal incidence, all measurements are carried out with unpolarized light. (c) Interferograms measured on the sample (red) and the reference (black) at 1,900 nm wavelength, showing phase shift corresponding to a negative index ofn=−0.93 (Δt=−1.68 fs). (d) Interferograms measured on the sample (red) and the reference (black) at 2,000 nm wavelength, showing a phase shift corresponding to an index of +0.65 (Δt=−0.52 fs). Multiple measurements gave an error in the time domain smaller than 0.2 fs corresponding to an index variation of less than±0.27. Figure 2: Interferometric measurements of the broken symmetry coupled nanorings. ( a ) Tilted-view scanning electron microscopy image of a metamaterial made of two aligned nanoring layers ( dx = dy =0 nm). The scale bar represents 500 nm. ( b ) Schematic of the Michelson interferometer. The metamaterial under test is made of two layers of nanorings, shifted with respect to each other ( dx = dy =L ). The thickness (index) of our metamaterial and reference is d meta ( n meta ) and d ref ( n ref ), respectively. The time delay between the two corresponding interferograms is related to the index of the metamaterial by n meta =1+ c 0 Δ t /2 d meta +( n ref −1) d ref / d meta ( Supplementary Fig. S6 ), where c 0 is the speed of light in vacuum. After planarization, the thickness of the metamaterial is d meta =110 nm and the thickness of the reference on the same substrate is d ref =80 nm ( n ref =1.5). The chess metamaterial being polarization independent at normal incidence, all measurements are carried out with unpolarized light. ( c ) Interferograms measured on the sample (red) and the reference (black) at 1,900 nm wavelength, showing phase shift corresponding to a negative index of n =−0.93 (Δ t =−1.68 fs). ( d ) Interferograms measured on the sample (red) and the reference (black) at 2,000 nm wavelength, showing a phase shift corresponding to an index of +0.65 (Δ t =−0.52 fs). Multiple measurements gave an error in the time domain smaller than 0.2 fs corresponding to an index variation of less than±0.27. Full size image To directly observe the induced negative index, we performed transmission phase measurements with a Michelson interferometer, shown in Fig. 2b . The idler of a femtosecond tunable optical parametric oscillator was used as light source. The pulse duration is 200 fs with a repetition rate of 80 MHz. Comparison of the time delay between the interferogram on the chess metamaterial and the interferogram on an unpatterned region of the substrate infers the additional phase, that is the refractive index of the metamaterial [26] ( Supplementary Fig. S6 ). Measured interferograms at the excitation wavelengths of 1,900 and 2,000 nm, obtained from the chess metamaterial with shifts dx = dy =300 nm and a spacer thickness of s =50 nm, are presented in Fig. 2c . The temporal shift between the reference and the metamaterial interferograms in Fig. 2c shows a negative index of −0.93 observed at 1,900 nm at the experimentally observed antisymmetric resonance ( Supplementary Fig. S7 ), whereas in Fig. 2d , an index of +0.65 is obtained at 2,000 nm. This is in very good agreement with the full-wave simulation where a negative index of −1 is obtained around ω − s =50 nm, shifted . The ambiguity between a phase lag and lead is overcome by comparison with simulations or by measuring continuously the delay from a point where the index is known ( Supplementary Fig. S8 ). We have thus directly observed, for the first time, negative index in a metamaterial made of negatively coupled closed-ring structures. The assignment of an index to a thin film has been subject to debate and is justified by the possibility to explain the optical observables by the retrieved effective paramaters [26] , [27] . Symmetry-dependent hybridization The influence of spatial symmetry breaking and the properties of the chess metamaterials can be further understood by analysing the optical transmission spectra of the coupled nanorings. 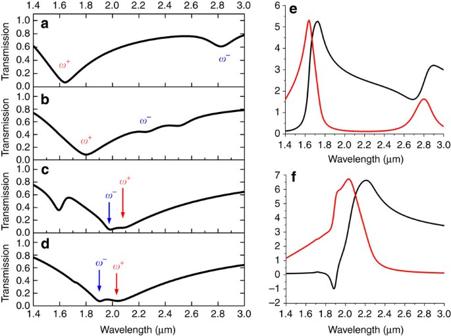Figure 3: Evolution of the transmission spectrum for two layer of coupled nanorings for different value of shift. In each case, one of the rings is shifted with respect to the other ring by an amountwithdx=dy=shift. (a) Shift=0. (b) Shift=L/3. (c) Shift=2L/3. (d) Shift=L. The blue shift of the antisymmetric mode and the red shift of the symmetric mode are clearly observed. An initial positive coupling between the nanorings (shift=0) becomes negative in the shifted configuration (shift=L). Higher order modes observed in the spectrum are discussed inSupplementary Fig. S1. (e) Effective index (real part in black and imaginary part in red) when the nanorings are aligned: the index is always positive. (f) Effective index (real part in black and imaginary part in red) when the nanorings are fully shifted: a negative index appears around the antisymmetric mode due to the spectral overlap of the symmetric and antisymmetric modes. Figure 3a shows calculated spectra for the case of a thin interlayer ( s =50 nm), with aligned ( dx = dy =0 nm) nanorings. In this case, the hybridization of the nanorings is normal and the antisymmetric mode occurs at longer wavelength (lower frequencies) than the symmetric mode, ω − s =50 nm, aligned < ω + s =50 nm, aligned , indicating a positive coupling between the rings. When the shift is increased ( Fig. 3b ), the two modes converge towards each other and spectrally cross ( Fig. 3c ). Figure 3d shows a metamaterial with lateral shifts of dx = dy =L. We observe drastic change compared with the normal hybridization picture. In this regime, the antisymmetric mode instead occurs at a shorter wavelength (higher frequencies), ω − s =50 nm, shifted > ω + s =50 nm, shifted . The relative spectral position of the symmetric ( ω + s =50 nm, shifted ) and antisymmetric ( ω − s =50 nm, shifted ) modes in the case of a shift of L is thus inverted, showing a negative coupling between the two nanorings due to the symmetry breaking [28] . The change in the sign of the coupling between the nanorings corresponds to a crossing of the real parts of the eigenfrequencies, and therefore leads to the spectral overlap between the antisymmetric and symmetric modes. The charge and electromagnetic fields distributions at each of the bonding and antibonding resonances are numerically analysed and presented in Supplementary Fig. S1 . Figure 3e shows an always positive index for aligned rings, whereas a negative-index region occurs in Fig. 3f for a full shift. The additional resonances in Fig. 3 , correspond to the hybridization of higher order multipoles of the rings [29] . Near-field patterns at these resonances are presented in Supplementary Fig. S1 . Figure 3: Evolution of the transmission spectrum for two layer of coupled nanorings for different value of shift. In each case, one of the rings is shifted with respect to the other ring by an amount with dx = dy =shift. ( a ) Shift=0. ( b ) Shift= L /3. ( c ) Shift=2 L /3. ( d ) Shift= L . The blue shift of the antisymmetric mode and the red shift of the symmetric mode are clearly observed. An initial positive coupling between the nanorings (shift=0) becomes negative in the shifted configuration (shift= L ). Higher order modes observed in the spectrum are discussed in Supplementary Fig. S1 . ( e ) Effective index (real part in black and imaginary part in red) when the nanorings are aligned: the index is always positive. ( f ) Effective index (real part in black and imaginary part in red) when the nanorings are fully shifted: a negative index appears around the antisymmetric mode due to the spectral overlap of the symmetric and antisymmetric modes. Full size image The evolution of the index of refraction for two layers of nanorings with symmetry breaking revealed an always positive refractive index for the aligned nanorings ( dx = dy =0), whereas a negative-index region is obtained when there is sufficient shift between the strongly coupled nanorings ( Fig. 3 ). The emergence of optical negative index in this metamaterial stems from the spectral overlap of symmetric and antisymmetric modes, corresponding to electric and magnetic dipole moments, respectively. In the negative coupling regime, the long-lived resonance (antisymmetric mode) occurs at higher energy than the short-lived resonance (symmetric mode). The modes can thus naturally overlap because the second resonance (antisymmetric mode) occurs in the broad negative tail (strongly coupled to far field) of the first resonance (symmetric mode) leading to negative refractive index. In the case of aligned resonators (positive coupling), the modes are difficult to overlap, which leads to positive index or a single negative medium [5] , [22] . Any attempt to build 3D metamaterials from those systems leads to a bandgap instead of a negative-index passband ( Supplementary Figs S9 and S10 ). We shall demonstrate that a medium built from such negatively coupled discrete plasmonic particles will support backward propagating waves. Three-dimensional chess metamaterials A multilayer of the chess metamaterial, exclusively exploiting localized resonances, leads to the tight coupling and the Fano-type interferences between those multiple localized modes. This results in the formation of an ultra-broad negative index band. 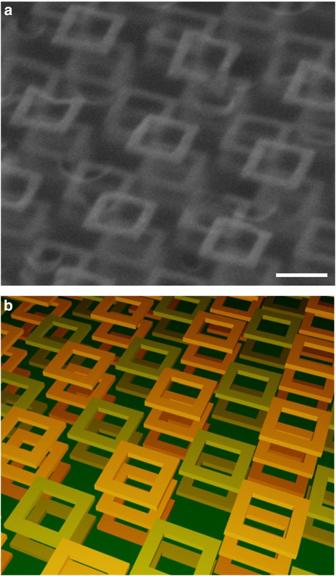Figure 4: SEM of the 3D chess metamaterial structure. (a) Tilted-view electron micrograph of the 3D structure (ten layers) of stacked broken symmetry nanorings fabricated by stacked electron beam lithography. The scale bar represents 250 nm. The structure consists of layers of nanorings separated by an insulator (SU-8). Each layer of nanorings is shifted with respect to the adjacent layer. The dimensions of the rings are: period=600 nm,L=300 nm,w=60 nm,t=30 nm,s=50 nm. The last layer is also covered by SU-8. (b) Sketch of the corresponding metamaterial. Figure 4 shows the fabricated 3D chess metamaterial consisting of ten-layer closed ring and spacer. The symmetry is laterally broken by shifting each layer with respect to the adjacent ones. The transmission spectra of the 3D chess metamaterials with different numbers of fabricated gold nanoring layers, from two to five, are calculated using finite-difference time domain numerical simulations ( Fig. 5a ). Measurement results are shown in Fig. 5b , and good agreement with calculations is found. By stacking the shifted nanorings, a passband builds up between the wavelengths of 1.3 and 2.3 μm. This extremely broad passband constitutes the negative-index region originating from the negative coupling between the nanorings ( Supplementary Fig. S11 ). The negative index can be interpreted as resulting from Fano resonances or the spectral overlap between resonant modes of opposite symmetry. These modes interact with the incident light continuum and contribute to the effective permittivity and the permeability. The strategy presented here, consisting of overlapping spectrally localized resonances can thus be regarded as a negative index originating from Fano resonances. 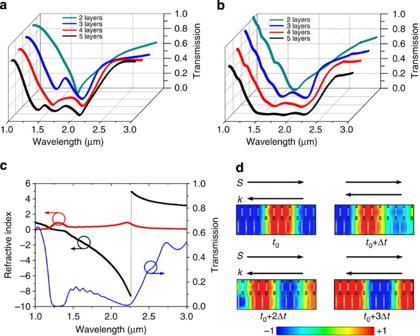Figure 5: Dispersion of the 3D chess metamaterial. (a) Simulated transmission spectra for different numbers of ring layers from two to five. (b) Measured transmission spectra for different numbers of metamaterial layers. Good agreement between experiment and theory is found. Here the last layer in each case is covered by 80 nm of SU-8. A slightly smaller transmission measured in experiment is attributed to deviations from the ideal structure, as seen inFig. 4a. The formation of the passband between 1.3 and 2.3 μm can be observed. The low transmission in experiment with increasing number of layers is due to fabrication imperfection. (c) Effective metamaterial index and transmission calculated for 20 layers of nanorings. Because the structure is constructed from coupled resonances, phase ambiguities arise in the determination of the index of refraction due to rapid phase rotation30,31. Detailed simulations using equivalent thin film of the metamaterial were used for branch selection. The black and red curves (left axis) are the real and imaginary parts of the effective refractive index and demonstrate low-loss operation over a broad frequency range. The blue curve (right axis) is the transmission of the corresponding metamaterial. The index is negative in the entire ‘Fano-induced’ passband of 1.3–2.3 μm. (d) Time evolution of uniform phase fronts (normalized electric field) in the bulk metamaterial showing backward waves atλ=1.6 μm (time increases from left to right and top to bottom).Sandkare the poynting vector and wavevector, respectively, and are antiparallel in the negative-index region. Figure 5c shows the effective refractive index of the metamaterial made of 20 layers of metallic nanorings, which is unambiguously determined by replacing the metamaterial with a thin film model [30] , [31] . The figure of merit (FOM) is an important parameter of negative-index metamaterials and is simply defined as FOM=| n ′/ n″ | where n ′ and n″ are the real and imaginary parts of the index. For a bulk metamaterial structure made of twenty ring layers presented in Fig. 5c , we found an FOM of ~10 at 2 μm ( Supplementary Fig. S12 ). The broadband and low-loss operation can also be observed from the real and imaginary parts of the index of refraction. In thin metamaterials, the localized modes reradiate in free space and the radiation loss is high. In thicker samples, the loss is decreased because the radiation from different rings cancelled inside the structure when they are out of phase, leading to decreased radiation loss of the bulk metamaterial. Figure 5d shows the time evolution of the wave inside the metamaterial structure at the middle of the passband, demonstrating the backward waves in a bulk metamaterial made of a single type of discrete resonators. Movies of the time evolution of wavefronts in the metamaterial in negative- and positive-index regions are presented in Supplementary Movies 1–6 . Moreover, phase measurements on the multilayer metamaterial, using a broadband Mach–Zehnder interferometer, confirm the broadband nature of our structure ( Supplementary Fig. S8 ). We have however not fabricated the 20 layers of rings to observe the full bandwidth (~1 μm) of the system. We would like to note that the assignment of effective index to our structure is justified by the single-mode operation in the region of interest, but, the index presented here is only valid for near normal incidence, when the in-plane wavevector is much smaller than the in-plane reciprocal lattice vector of the metamaterial. The transition in the real part of the index is also observed in the fishnet structure [32] , and alternative methods for retrieval have been discussed elsewhere [33] . In our structure, it originates from a transition from a negative-index mode to a positive index mode governing propagation in the system ( Supplementary Figs S13 and S14 ). Interestingly, wavefronts are uniformly distributed in our metamaterial unlike the fishnet system, where light was mainly travelling through the air holes [15] . Our strategy, as a fully discrete particle route, is thus a possible path toward 3D isotropic optical metamaterials [34] , [35] , [36] . It is worth noting that symmetry breaking, despite being considered in the context of Fano resonances, has never been used to create a complex effective medium (see ref. 37 and references therein), and particularly a negative-index medium operating at optical frequency. Figure 4: SEM of the 3D chess metamaterial structure. ( a ) Tilted-view electron micrograph of the 3D structure (ten layers) of stacked broken symmetry nanorings fabricated by stacked electron beam lithography. The scale bar represents 250 nm. The structure consists of layers of nanorings separated by an insulator (SU-8). Each layer of nanorings is shifted with respect to the adjacent layer. The dimensions of the rings are: period=600 nm, L =300 nm, w =60 nm, t =30 nm, s =50 nm. The last layer is also covered by SU-8. ( b ) Sketch of the corresponding metamaterial. Full size image Figure 5: Dispersion of the 3D chess metamaterial. ( a ) Simulated transmission spectra for different numbers of ring layers from two to five. ( b ) Measured transmission spectra for different numbers of metamaterial layers. Good agreement between experiment and theory is found. Here the last layer in each case is covered by 80 nm of SU-8. A slightly smaller transmission measured in experiment is attributed to deviations from the ideal structure, as seen in Fig. 4a . The formation of the passband between 1.3 and 2.3 μm can be observed. The low transmission in experiment with increasing number of layers is due to fabrication imperfection. ( c ) Effective metamaterial index and transmission calculated for 20 layers of nanorings. Because the structure is constructed from coupled resonances, phase ambiguities arise in the determination of the index of refraction due to rapid phase rotation [30] , [31] . Detailed simulations using equivalent thin film of the metamaterial were used for branch selection. The black and red curves (left axis) are the real and imaginary parts of the effective refractive index and demonstrate low-loss operation over a broad frequency range. The blue curve (right axis) is the transmission of the corresponding metamaterial. The index is negative in the entire ‘Fano-induced’ passband of 1.3–2.3 μm. ( d ) Time evolution of uniform phase fronts (normalized electric field) in the bulk metamaterial showing backward waves at λ =1.6 μm (time increases from left to right and top to bottom). S and k are the poynting vector and wavevector, respectively, and are antiparallel in the negative-index region. Full size image We reported the first experimental demonstration of an ultra-broadband-negative index in bulk optical metamaterials by controlling the symmetries of 3D localized plasmonic resonances using discrete closed metallic nanorings. A 3D, polarization-independent, negative-index metamaterial using one type of meta-atom at optical frequencies in a ‘Fano-induced negative index’ approach has been reported. We have broken the paradigm of negative index with closed nanorings. The ability to manipulate light with the spatial symmetry of 3D coupled metallic nano-particles may enable a new era in the design of metamaterials, opening the way to the observation of complex topological effects. We have also overcome the problem of current optical negative-index metamaterials (based on infinitely long metallic components) as plasmonic wave-guiding systems (fishnet and coupled coaxial waveguides, for example) that are inherently 2D and thus insufficient to realize 3D isotropic metamaterials, but our structure is still angular dependant. The exclusive use of localized plasmonic modes should allow the design of angle-independent metamaterials and pave the way towards low-loss linear and non-linear metamaterials (where symmetries have a fundamental role), novel designs of microwave, terahertz and optical meta-plasmonic devices. Sample fabrication The samples were fabricated by stacked electron beam lithography. The 30-nm-thick first-ring layer and the alignment marks are patterned on a 4-nm-thick indium tin oxide film coated on a glass substrate by EBL (electron beam lithography, CRESTEC CABL-9,510CC). The lithography is followed by e-beam evaporation of gold (Solution, CHA Industries) and lift-off process. The 80-nm-thick interlayer made of SU-8 2000.5 (Microchem Corp.) is diluted by a thinner solvent (Cyclopentanon), spun over the first-ring layer, cross-linked by UV light exposure, and baked on a hot plate. The thickness of the interlayer can be controlled by changing the ratio between SU-8 2000.5 and the solvent as well as the spinning speed. Because of the very low viscosity of the interlayer, the surface of the interlayer is automatically planarized and the distance between the ring layers is 50 nm after 95 °C baking on a hot plate. The fabrication is repeated using alignment marks of adjacent layers until the obtainment of the 3D chess metamaterial. Optical measurements The transmission spectra are measured using a Brucker instrument Fourier transform infrared spectrometer equipped with a Cassegrain objective. The near-infrared illumination is focused on the 30 × 30 μm 2 samples. The sample area is filtered using an aperture. The transmitted signal is collected by another microscope objective on to a liquid nitrogen-cooled mercury-cadmium-telluride detector. In the measurement of Fig. 2 , using the Michelson interferometer, the thickness of the metamaterial is d meta =110 nm and the thickness of the reference SU-8 just beside the structure is d ref =80 nm ( Supplementary Fig. S6 ). The time delay between the two interferograms on the sample and on the reference is given by: Δ t =2 d meta n meta / c 0 −[2 d ref n ref / c 0 −2( d meta − d ref )/ c 0 ] and thus: n meta =1+ c 0 Δ t /2 d meta +( n ref −1) d ref / d meta . Phase measurements of the multilayer metamaterial are performed using a broadband Mach–Zehnder interferometer coupled to a spectrometer, and capable of providing the broadband phase response in a single measurement ( Supplementary Fig. S8 ). Numerical simulations Numerical simulations of the chess metamaterial are carried out using a FDTD (finite-difference time domain) package (CST Microwave Studio). The periodic systems are modelled using their unit cells with periodic boundary conditions. The theoretical effective parameters are calculated from numerical simulation results using an inversion algorithm. How to cite this article: Kanté, B. et al. Symmetry breaking and optical negative index of closed nanorings. Nat. Commun. 3:1180 doi: 10.1038/ncomms2161 (2012).